The thermodynamic patterns of eukaryotic genes suggest a mechanism for intron–exon recognition The essential cis - and trans -acting elements required for RNA splicing have been defined, however, the detailed molecular mechanisms underlying intron–exon recognition are still unclear. Here we demonstrate that the ratio between stability of mRNA/DNA and DNA/DNA duplexes near 3′-spice sites is a characteristic feature that can contribute to intron–exon differentiation. Remarkably, throughout all transcripts, the most unstable mRNA/DNA duplexes, compared with the corresponding DNA/DNA duplexes, are situated upstream of the 3′-splice sites and include the polypyrimidine tracts. This characteristic instability is less pronounced in weak alternative splice sites and disease-associated cryptic 3′-splice sites. Our results suggest that this thermodynamic pattern can prevent the re-annealing of mRNA to the DNA template behind the RNA polymerase to ensure access of the splicing machinery to the polypyrimidine tract and the branch point. In support of this mechanism, we demonstrate that RNA/DNA duplex formation at this region prevents pre-spliceosome A complex assembly. RNA splicing is coupled with transcription and catalysed by a spliceosome nucleoprotein complex that acts to remove introns and re-join exonic sequences [1] . This process involves recognition of the 5′-splicing sites by U1 snRNPs [2] , [3] (small nuclear ribonucleoproteins). The 3′-inron–exon boundary recognition requires SF1 to interact with the branch point (BP) sequence [4] , [5] ; U2AF65 [6] (ref.6) with the polypyrimidine tract (PPT) and U2AF35 with the 3′-splice site [6] , [7] . U2AF recruit the U2 snRNP, which replaces SF1 to bind the BP and catalyses exon re-joining [7] . Although all these steps have been intensively studied, the detailed mechanisms underlying recognition of such degenerative sequences as the BP and PPT are still unclear. This raises the question whether exonic and intronic sequences are endowed with other attributes that can contribute to intron–exon recognition. As it reads the information encoded throughout the genome, RNA polymerase II can travel along the DNA template for thousands of nucleotides. In the process, it encounters the physical forces of DNA/DNA and RNA/DNA pairing that can vary depending on the local sequence composition. It has been shown [8] , [9] , [10] that the 5′- and 3′-untranslated regions (UTRs), introns and exons have characteristic guanine/cytosine (GC) content, which could affect RNA transcription and processing. Nucleotide composition could influence protein recruitment [9] , RNA secondary structure [10] , transcription rate [11] , [12] , DNA melting [13] or RNA/DNA and DNA/DNA duplex stability [14] . The free energy (ΔG) necessary to unwind polynucleotide duplexes with defined length can be calculated from the measured values of entropy (ΔS) and enthalpy (ΔH) for the 10 possible nearest-neighbour DNA/DNA [15] , [16] , [17] , [18] , [19] , [20] interactions, and the 16 possible RNA/DNA [21] , [22] interactions. We have previously shown that exons possess more stable RNA/DNA duplexes than introns in Saccharomyces cerevisiae [14] . However, our original approach did not allow for direct comparisons between the stability of RNA/DNA and DNA/DNA duplexes because the ΔS and ΔH parameters used for DNA/DNA duplexes [19] lead to overestimation of its ΔG in comparison with ΔG of RNA/DNA duplexes. This work aims to study the role of thermodynamic stability in RNA splicing by using appropriate thermodynamic parameters that allow comparison of mRNA/DNA with DNA/DNA duplex stability. We demonstrate that throughout transcripts, the most unstable mRNA/DNA duplexes, compared with the corresponding DNA/DNA duplexes, are situated upstream of the 3′-splice sites. Our results suggest that this thermodynamic pattern can prevent the re-annealing of mRNA to the DNA template to ensure access of the splicing machinery to the PPT. Thermodynamic stability of RNA/DNA versus DNA/DNA duplexes To evaluate if the measured nearest-neighbour parameters permit accurate comparison between thermodynamic stability of RNA/DNA and DNA/DNA duplexes, we performed high-resolution measurement of the melting temperature (Tm) and compared it with the calculated mean value of ΔG for the nearest-neighbour interactions of RNA/DNA [22] and DNA/DNA [20] duplexes for three variants of the human IL2 gene [12] , namely wIL2 (27% GC content), natural IL2 (39% CG) and eIL2 (60% GC content). We found strong correlation (0.945 correlation coefficient, P =0.005) between the measured Tm and the calculated ΔG values ( Fig. 1a and Supplementary Fig. S1a ). Our results suggest that calculation of ΔG using these parameters allows for accurate comparison of the difference in thermodynamic stability between RNA/DNA and DNA/DNA duplexes. In addition, we confirm the prediction for large variations between DNA/DNA [20] and RNA/DNA duplex stability [22] . The DNA/DNA duplex of wIL2 is more stable (Tm=75.81 (C°) and ΔG=1.17 (kcal mol −1 )) in comparison with the respective RNA/DNA duplex (Tm=73.68 (C°) and ΔG=1.12 (kcal mol −1 )). In contrast, the RNA/DNA duplex of eIL2 is more stable (Tm=91.88 (C°) and ΔG=1.64 (kcal mol −1 )) than the respective DNA/DNA duplex (Tm=90.31 (C°) and ΔG=1.51 (kcal mol −1 )). To further evaluate the variation between RNA/DNA and DNA/DNA duplex stability, we performed high-resolution melting analysis of another variant of the IL2 gene [12] called eIL2-IL2. Half of the eIL2-IL2 sequence is identical to the corresponding sequence of eIL2 (60% GC content) and the other half originates from IL2 (39% CG). Remarkably, both RNA/DNA and DNA/DNA duplexes dissociate in two steps as a result of the big difference between the thermodynamic stability of the eIL2 part and the IL2 part of the eIL2-IL2 gene ( Supplementary Fig. S1b ). Moreover, the DNA/DNA duplex of the IL2 part is more stable (Tm=80.7 (C°)) in comparison with the same RNA/DNA duplex (Tm=77 (C°)). In contrast, the DNA/DNA duplex of the eIL2 part is less stable (Tm=87.5 (C°)) in comparison with the corresponding RNA/DNA duplex (Tm=88.9 (C°)). The observed change in the melting behaviour of RNA/DNA and DNA/DNA duplexes in the context of the same molecule further supports the finding that nucleotide composition can change the ratio of the thermodynamic stability of RNA/DNA to DNA/DNA duplexes. Hereafter, we will refer to the difference between the ΔG of DNA/DNA and the ΔG of RNA/DNA duplexes as stability bias (ΔG bias). Regions with higher stability of the RNA/DNA duplex than the corresponding DNA/DNA duplex will be referred to as ‘RNA/DNA biased’, and regions with higher stability of the DNA/DNA duplex in comparison with RNA/DNA duplexes as ‘DNA/DNA biased’. 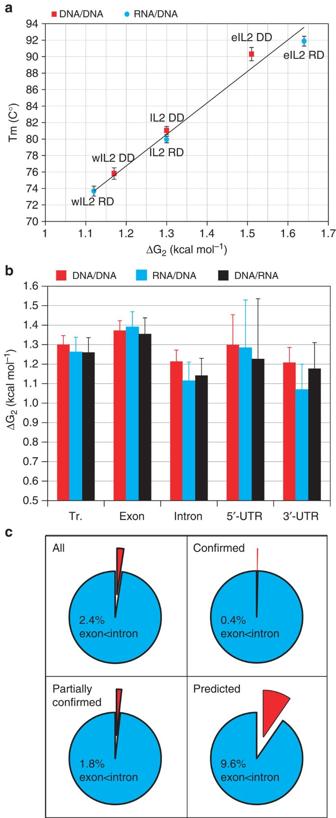Figure 1: Thermodynamic properties of the transcripts. (a) Correlation between ΔG and Tm of DNA/DNA and RNA/DNA duplexes of wIL2, IL2 and eIL2 gene variants. All experiments are performed in triplicates and the error bars represent the s.e.m. The window size for ΔG calculations is indicated with subscript number after ΔG. (b) Mean values of ΔG of DNA/DNA (DD), sense RNA/DNA (RD) and antisense RNA/DNA (DR) duplexes of annotated 5′-UTRs, exons, introns and 3′-UTRs of allC. eleganstranscripts. The error bars represent s.d. (c) Fraction of the transcripts with more stable RNA/DNA duplexes in introns compared with exons, for all transcript types or broken down by validation status—confirmed, partially confirmed and predicted transcripts. Figure 1: Thermodynamic properties of the transcripts. ( a ) Correlation between ΔG and Tm of DNA/DNA and RNA/DNA duplexes of wIL2, IL2 and eIL2 gene variants. All experiments are performed in triplicates and the error bars represent the s.e.m. The window size for ΔG calculations is indicated with subscript number after ΔG. ( b ) Mean values of ΔG of DNA/DNA (DD), sense RNA/DNA (RD) and antisense RNA/DNA (DR) duplexes of annotated 5′-UTRs, exons, introns and 3′-UTRs of all C. elegans transcripts. The error bars represent s.d. ( c ) Fraction of the transcripts with more stable RNA/DNA duplexes in introns compared with exons, for all transcript types or broken down by validation status—confirmed, partially confirmed and predicted transcripts. Full size image Thermodynamic properties of Caenorhabditis elegans genome To explore the possible role of the thermodynamic properties of the DNA/DNA and RNA/DNA duplexes, we calculated their corresponding ΔG values throughout the entire genome of C. elegans using the measured nearest-neighbour parameters [20] , [22] and a sliding-window approach [23] with 1 bp step and window size of 2 bp. The results revealed a striking correlation between the mean value of ΔG for exons, introns, 5′-UTRs, 3′-UTRs and transcripts ( Fig. 1b ). On average, the exonic sequences are more stable than 3′-UTRs and intronic sequences ( Fig. 1b ). Remarkably, 97.6% of the transcripts possess more thermodynamically stable RNA/DNA duplexes in exonic sequences in comparison with the corresponding intronic sequences ( Fig. 1c ). For the transcripts classified as ‘confirmed’, the correlation was even more compelling, with only 43 out of 10,960 (0.4%) having higher RNA/DNA duplexes stability in their intronic sequences. However, for transcripts classified as ‘predicted’ higher intronic compared with exonic RNA/DNA duplexes, stability was over 20 times more frequent (401 out of 4,167, or 9.6%) than in the ‘confirmed’ group, which may indicate false-positive transcript predictions. This suggests that the thermodynamic parameters can be useful in refining de novo gene structure prediction in C. elegans . Particularly interesting was the observed strong DNA/DNA bias in intronic sequences contrasting with the absence of bias in exonic sequences ( Fig. 1b ). To map the regions in transcripts that contribute to differential stability, we calculated the thermodynamic profile of the 50 bp upstream and the 50 bp downstream of the transcript start sites, the 5′- and 3′- splice sites and the ends of the 3′-UTRs of all C. elegans transcripts ( Fig. 2a ). This approach allows alignment and colour-coded representation of the thermodynamic profile of the individual sequences with respect to the regions responsible for RNA processing ( Fig. 2 ). As the RNA polymerase maintains a 9-bp RNA/DNA duplex in the transcription bubble during elongation, we used a window size of 9 bp for ΔG calculations. In addition to the observation that introns are less stable than exons ( Fig. 2a and Supplementary Fig. S2 ), we found that the least stable RNA/DNA duplex is located upstream of the 3′-splice site, and includes the polyU tract [24] characteristic of the 3′-consensus in C. elegans ( Fig. 3 ). This region is directly followed by a more stable region, which includes the 3′-splice site. At the 5′-splice site, a more stable region at the exon–intron boundary is followed by an intronic region with a significantly lower RNA/DNA duplex stability ( Fig. 2a ). The pattern is similar, but not as pronounced, for DNA/DNA duplex stability of the same sequences ( Fig. 2a ). As a result, the DNA/DNA bias is most significant at both intron ends ( Fig. 2d and Supplementary Fig. S3a ). Remarkably, next to these regions are situated the regions with the strongest RNA/DNA bias, which include the 5′- and 3′-splice sites. 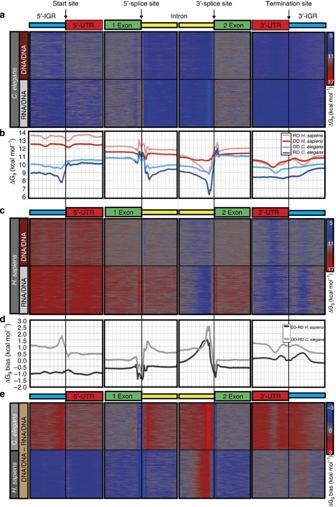Figure 2: A pattern of thermodynamic stability forC. elegans and H. sapienstranscripts. (a) Intensity plot of ΔG of DNA/DNA and RNA/DNA duplexes of the 50-bp sequences surrounding: all annotated start sites, 5′- and 3′-splice sites of 40,000 exon–intron–exon units and all annotated 3′-UTR ends ofC. eleganstranscripts. (b) Mean values of ΔG of DNA/DNA and RNA/DNA duplexes of the 50-bp sequences surrounding: all annotated start sites, 5′- and 3′-splice sites of 40,000 exon–intron–exon units, and all annotated 3′-UTR ends ofC. elegansandH. sapienstranscripts. (c) Intensity plot of ΔG of DNA/DNA and RNA/DNA duplexes of the 50 bp sequences surrounding: all annotated start sites, 5′- and 3′-splice sites of all exon–intron–exon units of chromosome 1, and all annotated 3′-UTR ends ofH. sapienstranscripts. (d)Mean values of the ΔG bias of the 50-bp sequences surrounding: annotated start sites, 5′- and 3′-splice sites, and the ends of the 3′-UTR of allC. elegansandH. sapienstranscripts. (e) Intensity plot of the ΔG bias of the 50-bp sequences surrounding: the annotated start sites ofC. elegansandH. sapienstranscripts, the annotated ends of the 3′-UTR ofC. elegansandH. sapienstranscripts, the 5′- and 3′-splice sites of 40,000 exon–intron–exon units ofC. elegans, and the 5′-and 3′-splice sites of exon–intron–exon units of chromosome 1 ofH. sapienstranscripts. Figure 2: A pattern of thermodynamic stability for C. elegans and H. sapiens transcripts. ( a ) Intensity plot of ΔG of DNA/DNA and RNA/DNA duplexes of the 50-bp sequences surrounding: all annotated start sites, 5′- and 3′-splice sites of 40,000 exon–intron–exon units and all annotated 3′-UTR ends of C. elegans transcripts. ( b ) Mean values of ΔG of DNA/DNA and RNA/DNA duplexes of the 50-bp sequences surrounding: all annotated start sites, 5′- and 3′-splice sites of 40,000 exon–intron–exon units, and all annotated 3′-UTR ends of C. elegans and H. sapiens transcripts. ( c ) Intensity plot of ΔG of DNA/DNA and RNA/DNA duplexes of the 50 bp sequences surrounding: all annotated start sites, 5′- and 3′-splice sites of all exon–intron–exon units of chromosome 1, and all annotated 3′-UTR ends of H. sapiens transcripts. ( d )Mean values of the ΔG bias of the 50-bp sequences surrounding: annotated start sites, 5′- and 3′-splice sites, and the ends of the 3′-UTR of all C. elegans and H. sapiens transcripts. ( e ) Intensity plot of the ΔG bias of the 50-bp sequences surrounding: the annotated start sites of C. elegans and H. sapiens transcripts, the annotated ends of the 3′-UTR of C. elegans and H. sapiens transcripts, the 5′- and 3′-splice sites of 40,000 exon–intron–exon units of C. elegans , and the 5′-and 3′-splice sites of exon–intron–exon units of chromosome 1 of H. sapiens transcripts. 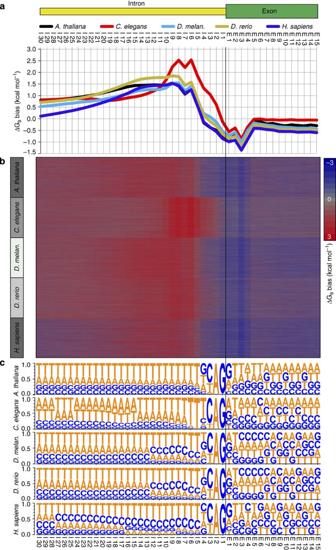Figure 3: Nucleotide distribution and thermodynamic patterns of 3′-splice sites of transcripts from different species. (a) Mean values of the ΔG bias surrounding the 3′-splice sites ofA. thaliana,C. elegans, D. melanogaster, D. rerioandH. sapienstranscripts. (b) Intensity plot of the ΔG bias of the sequences surrounding 3′-splice sites ofA. thaliana,C. elegans, D. melanogaster, D. rerioandH. sapienstranscripts. (c) Nucleotide distribution of the sequences surrounding the 3′-splice sites ofA. thaliana, C. elegans, D. melanogaster, (D). rerioandH. sapienstranscripts. The distance from the 3′-splice sites intron/exon junctions is specified under each position for the intronic (I) and exonic (E) regions. Full size image Figure 3: Nucleotide distribution and thermodynamic patterns of 3′-splice sites of transcripts from different species. ( a ) Mean values of the ΔG bias surrounding the 3′-splice sites of A. thaliana , C. elegans, D. melanogaster, D. rerio and H. sapiens transcripts. ( b ) Intensity plot of the ΔG bias of the sequences surrounding 3′-splice sites of A. thaliana , C. elegans, D. melanogaster, D. rerio and H. sapiens transcripts. ( c ) Nucleotide distribution of the sequences surrounding the 3′-splice sites of A. thaliana, C. elegans, D. melanogaster, (D). rerio and H. sapiens transcripts. The distance from the 3′-splice sites intron/exon junctions is specified under each position for the intronic (I) and exonic (E) regions. Full size image We considered the possibility that the observed pattern is a consequence of the fact that most exons contain protein-coding sequences that have specific sequence constraints. However, the same pattern was observed for the exon–intron–exon units in both protein-coding regions and UTRs of the coding genes ( Supplementary Fig. S4 ). Furthermore, we found no significant difference between protein-coding and non-coding genes (results not shown). Taken together, the observations above suggest that the specific pattern of thermodynamic stability distribution is related to RNA splicing, a process that occurs co-transcriptionally and can be directly affected by the thermodynamic stability of the DNA/DNA and RNA/DNA duplexes. This is further supported by the thermodynamic stability profile at the start sites of the transcripts ( Fig. 2a ). In C. elegans , the 5′-end of about 70% of the mRNAs is produced in a process called ‘trans splicing’, whereby the transcript gets spliced to a short ‘splice leader’ RNA in a process similar to normal intron removal [25] ( cis -splicing). We found that the start sites of the trans -spliced transcripts have the characteristic thermodynamic profile of a 3′-splice site ( Fig. 2a and Supplementary Fig. S5 ), and differ from the conventional transcript start sites ( Supplementary Fig. S6 ). The identical thermodynamic properties of cis and trans 3′-splice sites suggest that they could contribute to the mechanism of RNA splicing. Thermodynamic stability pattern of eukaryotic transcripts To assess whether the observed thermodynamic stability patterns exist in mammals, we calculated the free energy near the splice sites in the human genome ( Fig. 2b ). In human transcripts, both RNA/DNA and DNA/DNA duplexes are more stable compared with C. elegans ( Fig. 2a–c ). The second difference observed is that human transcripts are RNA/DNA biased, except the regions upstream of the 3′-splicing sites and the 3′-UTRs. Moreover, we found that the 5′-UTRs of human transcripts are extremely stable. We analysed all first and second exon pairs that fall into 5′-UTRs. The thermodynamically stable region includes the first exon of the 5′-UTR and propagates to the intronic sequence, but does not reach the 3′-part of the intron and the second exon, even though it is also part of the 5′-UTR ( Supplementary Figs S7 and S8 ). It is known that the first exon and intron of genes possess specific features compared with the rest of the exon–intron pairs, such as shorter exon length [26] , longer intron length [27] and characteristic DNA methylation [28] and histone-modification profiles [29] . However, the relationship between these characteristics and the higher stability of the first exon and intron and the biological significance of these correlations are still unclear. Despite these differences, the thermodynamic profiles for Homo sapiens and C. elegans share three important features. First, the region of lowest RNA/DNA duplex stability within the transcript is situated in intronic sequences upstream of 3′-splice sites in both species ( Fig. 2a–c ). Second, this region possesses the strongest DNA/DNA bias ( Fig. 2a–c and Supplementary Fig. S3b ). Third, the 3′- and 5′-splice sites have the strongest RNA/DNA bias. Similar to C. elegans , in H. sapiens these patterns are observed in both coding and non-coding genes (results not shown) and in coding and UTRs of the coding genes ( Supplementary Fig. S7 ), supporting the idea that the observed profiles are linked to a transcription-coupled process. To check whether the observed thermodynamic stability patterns are evolutionarily conserved, we calculated ΔG near the splice sites of the plant Arabidopsis thaliana , the insect Drosophila melanogaster and the fish Danio rerio ( Supplementary Figs S9 and S10 ). The same trend as in C. elegans and H. sapiens was detected in those species ( Fig. 3 and Supplementary Figs S9 and S10 ), whereby the region of strongest DNA/DNA bias was situated within intronic sequences upstream of the 3′-splice sites. With the exception of H. sapiens , the full lengths of intronic sequences of all studied organisms were DNA/DNA biased. In contrast, the strongest RNA/DNA bias throughout the entire pool of measured transcripts was detected at the 3′- and 5′-splice sites of all species. These patterns are statistically significant with P -value <2e-15 (Methods). We found that the PPT, a degenerative, pyrimidine-rich sequence, required for intron–exon recognition is situated in the region of strongest DNA/DNA bias. It is remarkable that regions with significant differences in nucleotide composition among species would possess such a uniform DNA/DNA bias ( Fig. 3a–c and Supplementary Fig. S10 ). Thermodynamic pattern near alternative splice sites Most primary transcripts in metazoans are subject to alternative splicing, whereby the same sequence can be an intron in one transcript and an exon in another [30] . We calculated the thermodynamic stability of all human intron/exon units with a known alternative 3′-splice sites up to 50 bp away from each other and sorted them by increasing distance between the two sites ( Fig. 4a–d ). By this approach, the specific pattern of strong DNA/DNA bias upstream of 3′-splice sites and RNA/DNA bias at the 3′-splice site can be clearly seen for both alternative splice sites when the distance between them is over eight nucleotides. ( Fig. 4d ). The characteristic RNA/DNA bias for the 5′-alternative slice sites are also detectable, although less pronounced than the profile near 3′-splice sites ( Fig. 4d ). Some alternative splicing events are subject of intensive cell type-specific regulation, which allows differential expression of the splice variants. However, a substantial fraction of the alternative splicing events result in low-abundance alternative transcripts without detectable biological function. Such minor transcript variants are believed to be a result of splicing of inefficient splice sites. If the thermodynamic stability profile near the splice sites has a role in the splicing reaction, the constitutive splicing sites will possess more pronounced biases in the thermodynamic profiles than alternative splice sites of low splicing efficiency. We compared the thermodynamic profile near the 3′-splice sites of human constitutive exons, retained introns, cassette (skipped) exons and 3′-alternative splice sites ( Fig. 5a and Supplementary Fig. S11 ). The cassette exons that are present in one but skipped in other transcripts of the same gene possess similar thermodynamic stability profiles as the constitutive exons ( Fig. 5b ). However, 3′-alternative splice exons possess lower DNA/DNA bias upstream of the 3′-splice sites compared with the constitutive exons. The difference is even stronger for the retained introns, in which, an intron is not removed from the mature transcript ( Fig. 5a and Supplementary Fig. S11 ). The retained introns are believed to be a result of recognition failure of the weak splice sites that flank the introns [31] . Those week splice sites could be a result of the low DNA/DNA bias of the region. To assess if there is a link between the thermodynamic stability and the alternative splice site usage, we compared the 10% of 3′-alternative splice sites with either the lowest (10th percentile) or the highest splicing levels (90th percentile) [32] . Our results reveal that the 3′-alternative splice sites with the lower splicing levels possess lower DNA/DNA bias upstream of the 3′-splice sites than the average 3′-alternative splice sites ( Fig. 5c and Supplementary Fig. S12 ). In contrast, the 3′-alternative splice sites with higher splicing level possess higher DNA/DNA bias than the average 3′-alternative splice sites. Even the cassette exons with the lower splicing levels possess significantly diminished DNA/DNA bias than the average cassette exons and constitutive exons ( Fig. 5d and Supplementary Fig. S13 ). We also studied the thermodynamic profile near the 3′-splice sites of 5′-alternative splice exons as a negative control ( Fig. 5e ). There was no difference in the thermodynamic profile near the 3′-splice sites of higher and lower splicing level of 5′-alternative splice exons. These results suggest that the DNA/DNA bias upstream of the 3′-splice sites could be involved in 3′-spice site recognition. 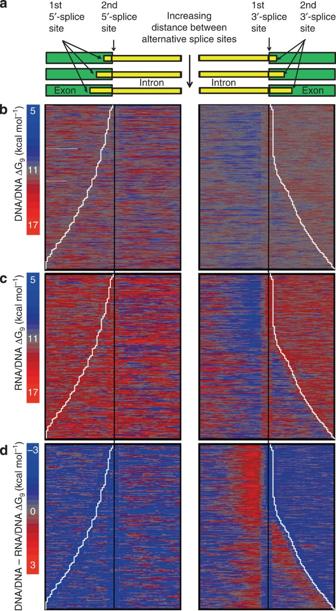Figure 4: Thermodynamic stability patterns of the 5′- and 3′-alternative splice sites inH. sapiens. (a) A scheme of the positioning of the 5′- and 3′- alternative splice sites in the intensity plots inb–d. (b) A plot of ΔG of DNA/DNA duplexes of the 50-bp sequences surrounding: all annotated alternative splice sites with <50 bp distance between them. The results for the 5′-splice sites are aligned with respect to the downstream 5′-alternative splice sites, indicated with a black line. The upstream 5′-alternative splice sites are indicated with a white line. The results for 3′-splice sites are aligned with respect to the upstream 3′-alternative splice sites, indicated with a black line. The downstream 3′-alternative splice sites are indicated with a white line. (c) A plot of ΔG of RNA/DNA duplexes of the 50-bp sequences surrounding: all annotated alternative splice sites with <50 bp distance between them. The results are aligned as indicated inb. (d) A plot of ΔG bias of the 50-bp sequences surrounding: the annotated alternative splice sites with <50 bp distance between them. The results are aligned as indicated inb. Figure 4: Thermodynamic stability patterns of the 5′- and 3′-alternative splice sites in H. sapiens . ( a ) A scheme of the positioning of the 5′- and 3′- alternative splice sites in the intensity plots in b – d . ( b ) A plot of ΔG of DNA/DNA duplexes of the 50-bp sequences surrounding: all annotated alternative splice sites with <50 bp distance between them. The results for the 5′-splice sites are aligned with respect to the downstream 5′-alternative splice sites, indicated with a black line. The upstream 5′-alternative splice sites are indicated with a white line. The results for 3′-splice sites are aligned with respect to the upstream 3′-alternative splice sites, indicated with a black line. The downstream 3′-alternative splice sites are indicated with a white line. ( c ) A plot of ΔG of RNA/DNA duplexes of the 50-bp sequences surrounding: all annotated alternative splice sites with <50 bp distance between them. The results are aligned as indicated in b . ( d ) A plot of ΔG bias of the 50-bp sequences surrounding: the annotated alternative splice sites with <50 bp distance between them. The results are aligned as indicated in b . 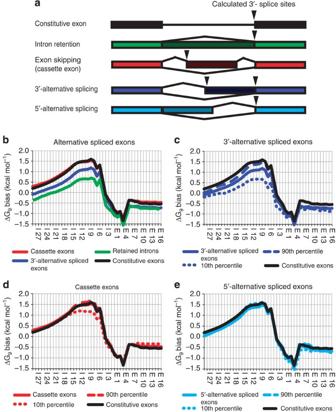Figure 5: Thermodynamic stability patterns of 3′-splice sites of the constitutively and alternatively spliced exons inH. sapiens. (a) A scheme of the alternative splicing events inb–d. The positions of the calculated sites are depicted by arrowheads. (b) Mean values of the ΔG bias across the sequences surrounding the 3′-splice sites of constitutive exons, cassette exons, 3′-alternative spliced exons and retained introns. The distance from the 3′-splice sites intronic/exon junctions is specified under each position for the intronic (I) and exonic (E) regions. (c) The mean value of the ΔG bias across the sequences surrounding the 3′-splice sites of 3′-alternative spliced exons and constitutive exons. 10th percentile is 10% of 3′-alternative splice sites with the lowest splicing level. 90th percentile is 10% of 3′-alternative splice sites with the highest splicing level. (d) Mean values of the ΔG bias across the sequences surrounding the 3′-splice sites of cassette exons and constitutive exons. (e) Mean values of the ΔG bias across the sequences surrounding 3′-splice sites of 5′-alternative spliced exons and constitutive exons. Full size image Figure 5: Thermodynamic stability patterns of 3′-splice sites of the constitutively and alternatively spliced exons in H. sapiens . ( a ) A scheme of the alternative splicing events in b – d . The positions of the calculated sites are depicted by arrowheads. ( b ) Mean values of the ΔG bias across the sequences surrounding the 3′-splice sites of constitutive exons, cassette exons, 3′-alternative spliced exons and retained introns. The distance from the 3′-splice sites intronic/exon junctions is specified under each position for the intronic (I) and exonic (E) regions. ( c ) The mean value of the ΔG bias across the sequences surrounding the 3′-splice sites of 3′-alternative spliced exons and constitutive exons. 10th percentile is 10% of 3′-alternative splice sites with the lowest splicing level. 90th percentile is 10% of 3′-alternative splice sites with the highest splicing level. ( d ) Mean values of the ΔG bias across the sequences surrounding the 3′-splice sites of cassette exons and constitutive exons. ( e ) Mean values of the ΔG bias across the sequences surrounding 3′-splice sites of 5′-alternative spliced exons and constitutive exons. Full size image Stability pattern near cryptic and authentic 3′-splice sites Metazoan transcripts contain large numbers of ‘cryptic’ splice sites that are inactivated due to suppression from nearby and advantageous authentic splice sites [33] . Mutation of the authentic splice sites activates the cryptic splice sites, leading to aberrant alternative splicing and frequently to genetic disease [34] , [35] . To understand how the thermodynamic profile can influence the splice site selection, we compared ΔG bias of disease-related cryptic 3′-splice sites [33] with their corresponding authentic splice sites. The cryptic splice sites can occur both upstream (in the intron) and downstream (in the exon) of the authentic 3′-splice site. We first analysed 21 cryptic 3′-splice sites situated more than 20 bp downstream from the authentic splice sites [33] ( Fig. 6a , Supplementary Fig. S14a and Supplementary Table S1 ). In this configuration, Pol II will transcribe first the authentic 3′-splice sites and then the cryptic 3′-splice sites. In this case, we do not see the characteristic region with the strongest DNA/DNA bias in front of the cryptic 3′-splice sites, which is present at the authentic 3′-splice sites. Such a pattern suggests that the absence of a DNA/DNA-biased sequence does not allow independent splicing events at cryptic 3′-splice sites. Mutation in the AG consensus of the authentic 3′-splice sites could still allow recognition of their upstream unstable regions by the spliceosome and finding of the AG consensus of the cryptic 3′-splice sites. 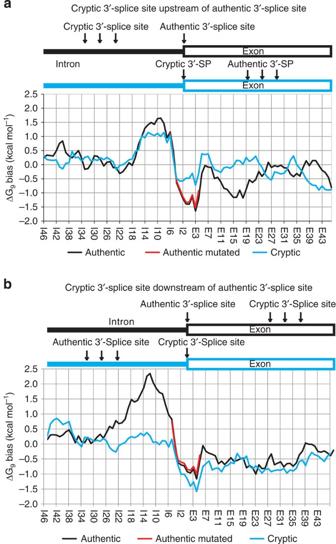Figure 6: Thermodynamic stability patterns of the cryptic 3′-splice sites inH. sapiens. (a) Mean values of the ΔG bias across the sequences, surrounding the authentic and the situated upstream cryptic 3′-splice sites. The distance from the 3′-splice sites intronic/exon junctions is specified under each position for the intronic (I) and exonic (E) regions. (b) Mean values of the ΔG bias across the sequences, surrounding authentic 3′-splice sites and corresponding cryptic 3′-splice sites located downstream from authentic 3′-splice. Figure 6: Thermodynamic stability patterns of the cryptic 3′-splice sites in H. sapiens. ( a ) Mean values of the ΔG bias across the sequences, surrounding the authentic and the situated upstream cryptic 3′-splice sites. The distance from the 3′-splice sites intronic/exon junctions is specified under each position for the intronic (I) and exonic (E) regions. ( b ) Mean values of the ΔG bias across the sequences, surrounding authentic 3′-splice sites and corresponding cryptic 3′-splice sites located downstream from authentic 3′-splice. Full size image We next analysed 15 cryptic sites situated more than 20 bp upstream of the authentic 3′-splice site [33] ( Fig. 6b , Supplementary Fig. S14b and Supplementary Table 2 ). In this configuration, Pol II together with the spliceosome factors will first encounter the cryptic 3′-splice sites and then the authentic splice sites. On average, the DNA/DNA bias is less pronounced at the region situated upstream of cryptic 3′-splice sites than at the same regions of the authentic splice sites. Furthermore, RNA/DNA bias is not as strong at cryptic 3′-splice sites as at authentic splice sites. Our results show that the characteristic thermodynamic profile of the 3′-splice sites is less pronounced in the cryptic 3′-splice sites, which could allow them to be bypassed by the Pol II without leading to a splicing event when the authentic splice site is functional. Thermodynamic profile of real exons and pseudoexons The BP sequence is a degenerative signal situated several nucleotides upstream of the PPT [36] . To map BPs in the context of the region of the strongest DNA/DNA bias, we calculated the free energy near 35 identified human BPs [37] Our results show that on average the BP is located upstream of the maximum DNA/DNA bias point but is still within the DNA/DNA bias region ( Fig. 7a ). 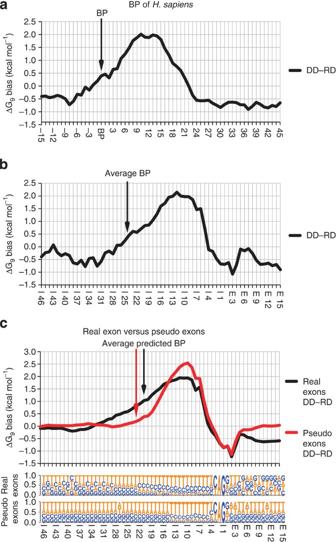Figure 7: Thermodynamic stability patterns near the 3′-splice sites and the BP of both real and pseudo exons inH. sapiens. (a) Mean values of the ΔG bias across the 50-bp sequences, surrounding the BP of 35 exons ofH. sapiens. The coordinates at the horizontal axis indicate the positions with respect of the BP. (b) Mean values of the ΔG bias across the 50-bp sequences, surrounding the 3′-splice sites of 35 exons ofH. sapiens. The average position of the BP is indicated. (c) Mean values of the ΔG bias across the 50-bp sequences surrounding the 3′-splice sites of both real and pseudo exons ofH. sapiens. The average position of the BP is indicated. DD, DNA/DNA; RD, sense RNA/DNA. Figure 7: Thermodynamic stability patterns near the 3′-splice sites and the BP of both real and pseudo exons in H. sapiens. ( a ) Mean values of the ΔG bias across the 50-bp sequences, surrounding the BP of 35 exons of H. sapien s. The coordinates at the horizontal axis indicate the positions with respect of the BP. ( b ) Mean values of the ΔG bias across the 50-bp sequences, surrounding the 3′-splice sites of 35 exons of H. sapien s. The average position of the BP is indicated. ( c ) Mean values of the ΔG bias across the 50-bp sequences surrounding the 3′-splice sites of both real and pseudo exons of H. sapien s. The average position of the BP is indicated. DD, DNA/DNA; RD, sense RNA/DNA. Full size image Pseudoexons are regions in the human genome flanked by sequences that resemble authentic splicing regulatory signals but are not spliced into mature mRNAs [38] , [39] , [40] . Previous work [39] has provided a reliable data set of such sequences [40] . We compared the thermodynamic stability near 3′-splice sites of the real non-coding exons and pseudoexons of the same data set ( Fig. 7c ). Although the maximum of the DNA/DNA bias was higher for the pseudoexons, this is likely due to the very stringent selection criteria for this data set, which would exclude over 25% of the known real exons. However, the high DNA-bias region was shorter for the 3′-splice sites upstream of the pseudoexonic sequences, which potentially puts it at a distance from the BP. To investigate this further, we compared the position of the potential BP in real exons and pseudoexons. As previously shown [39] , predicted BP consensus sequences are less frequently found in front of 3′-splice sites of pseudoexons. Predicted BP consensus sequences were only found for 56% of the pseudoexons, compared with 69% for the real exons. We found that, when present, the average predicted BP consensus sequences are located further away from the 3′-splice sites of pseudoexons in comparison with real exons ( Fig. 7c ). This, in combination with the short region with DNA/DNA bias, positions the predicted BP consensus sequences outside the DNA/DNA-biased region of the 3′-splice sites of pseudoexons ( Fig. 7c ). In contrast, the average predicted BP consensus sequence is situated inside the DNA/DNA-biased region of the 3′-splice sites of real exons ( Fig. 7c ), as was the case with experimentally confirmed BPs ( Fig. 7a ). Our results suggest that the positioning of BP consensus sequences outside the narrow DNA/DNA-biased regions of the 3′-splice sites can contribute to the absence of splicing in pseudoexons in addition to under-representation of the regulatory sequences [39] . All of the discussed results show that the elongating RNA polymerase, on its way through a DNA template, produces a RNA transcript with significant local differences in the potential for DNA/DNA and RNA/DNA duplex formation and unwinding, which are most pronounced near the 3′-splice sites. This characteristic instability is less pronounced in weak alternative splice sites and disease-associated cryptic 3′-splice sites, thus suggesting a role of the thermodynamic pattern for mRNA splicing. RNA/DNA annealing at DNA/DNA-biased regions impedes splicing It has recently been shown that depletion of two splicing factors, ASF/SF2 and RNPS1, which co-transcriptionally bind to the nascent mRNA, leads to formation of mRNA/DNA duplexes as a result of re-annealing of mRNA to DNA template strand in the wake of transcription [41] , [42] . The structure created by re-annealing of mRNA to DNA template is called R-loops [43] . The suppression of R-loop formation from splicing factors suggests that the re-annealing of mRNA to DNA template can interfere with proper RNA splicing [41] , [42] , [44] . Furthermore, Topo I topoisomerase, which removes negative supercoiling generated behind RNA polymerases during transcription, also suppresses R-loop formation [45] , [46] . The accumulation of negative supercoiling in Topo I-deficient cells is supposed to weaken DNA/DNA duplexes and facilitate both re-annealing of mRNA to the DNA template strand and R-loop formation. In the context of these findings, we propose that the detected DNA/DNA bias, upstream of the 3′-splicing site, prevents the re-annealing of mRNA after transcription to allow spliceosome assembling. To test this hypothesis, we studied whether the re-annealing of the RNA transcript to DNA in DNA/DNA-bias region, situated upstream of 3′-splice sites, can inhibit spliceosome assembling. In vitro experiments with crude nuclear extracts have demonstrated a stepwise assembling of the spliceosome onto RNA [47] , [48] , [49] . First, RNA is incorporated into a nonspecific heterogeneous nuclear ribonucleoprotein H complex that does not require ATP and functional splicing regulatory sequences. The addition of ATP leads to re-arrangement of RNA into a pre-spliceosomal complex A as a result of binding of U2AF65, U2AF35 and U2 snRNP to the PPT, 3′-splice sites and BP, respectively [47] , [50] . We studied whether the annealing of DNA oligonucleotides to RNA, near the 3′-spice site of exon 2 of AdML transcript, will influence the pre-spliceosome complex formation in crude nuclear extracts [51] , [52] . Our results show that the annealing of antisense DNA oligonucleotides covering the DNA/DNA-biased region and the BP region leads to inhibition of complex A formation ( Fig. 8 ) and partially impedes the formation of complex H. The same result was observed with an oligonucleotide covering the DNA/DNA-biased region alone. In contrast, the annealing of antisense DNA oligonucleotides to RNA at the 3′-splice site and the start of the exon does not influence complex A and H formation ( Fig. 8 ). The inhibition of complex A formation by annealing of DNA to the DNA/DNA-biased region further suggests that a strong DNA/DNA bias in this region is required to prevent the annealing of DNA to RNA to ensure spliceosome assembly. Such mechanism is also supported by the research of Krainer and collaborators [53] , who studied the splicing of SMN2 exon 7. They showed that the annealing of chimeric antisense oligonucleotides across the PPT sequence of the RNA of intron 6 leads to inhibition of splicing of exon 7 both in vivo and in vitro . 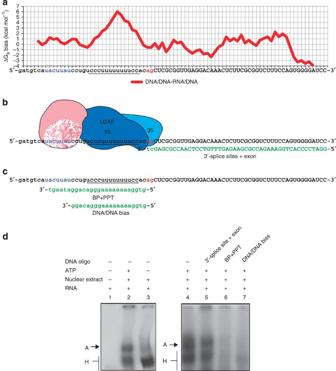Figure 8: Pre-spliceosome assembly onto the 3′-splice site of AdML RNA exon 2 with or without annealing of antisense DNA oligonucleotidesin vitro. (a–c) Schematic depiction of the experimental setup for the results shown ind. Black—AdML RNA transcript intron 1/exon 2 junction; lower case—intronic region, upper case—exonic region; blue—BP; underlined—PPT; red—3′-splice site; green—DNA antisense strand for either the splice site plus the exon, the BP+PPT, or the DNA/DNA-biased region. (a) The mean value of the ΔG bias surrounding the 3′-splice site of exon 2 of AdML promoter transcripts. (b) Pre-spliceosome A complex formation when antisense DNA oligonucleotide is annealed to exon 2 of AdML RNA. (c) Inhibition of the pre-spliceosome A complex formation when antisense DNA oligonucleotide is annealed to either the DNA/DNA-biased region plus the BP sequence or the DNA/DNA-biased region alone. (d) Spliceosome complex formation assay using HeLa nuclear extract. The pre-spliceosome complex A formation is not inhibited when antisense DNA oligonucleotide is annealed to both 3′-AG splice site and exonic sequence of AdML RNA (lane 5). The pre-spliceosome complex A formation is inhibited when an antisense DNA oligonucleotide is annealed to either the BP+PPT sequence (lane 6) or the DNA/DNA-biased region alone (lane 7). Figure 8: Pre-spliceosome assembly onto the 3′-splice site of AdML RNA exon 2 with or without annealing of antisense DNA oligonucleotides in vitro . ( a – c ) Schematic depiction of the experimental setup for the results shown in d . Black—AdML RNA transcript intron 1/exon 2 junction; lower case—intronic region, upper case—exonic region; blue—BP; underlined—PPT; red—3′-splice site; green—DNA antisense strand for either the splice site plus the exon, the BP+PPT, or the DNA/DNA-biased region. ( a ) The mean value of the ΔG bias surrounding the 3′-splice site of exon 2 of AdML promoter transcripts. ( b ) Pre-spliceosome A complex formation when antisense DNA oligonucleotide is annealed to exon 2 of AdML RNA. ( c ) Inhibition of the pre-spliceosome A complex formation when antisense DNA oligonucleotide is annealed to either the DNA/DNA-biased region plus the BP sequence or the DNA/DNA-biased region alone. ( d ) Spliceosome complex formation assay using HeLa nuclear extract. The pre-spliceosome complex A formation is not inhibited when antisense DNA oligonucleotide is annealed to both 3′-AG splice site and exonic sequence of AdML RNA (lane 5). The pre-spliceosome complex A formation is inhibited when an antisense DNA oligonucleotide is annealed to either the BP+PPT sequence (lane 6) or the DNA/DNA-biased region alone (lane 7). Full size image These results indicate that the DNA/DNA bias near 3′-splice sites influences the splicing process. However, the region of most pronounced DNA/DNA bias coincides with the PPT, which is known to be required for proper splicing [2] , [6] , [54] , [55] . This raises the question whether the PPT is required to ensure the DNA/DNA bias necessary to prevent the re-annealing of mRNA to DNA only or its degenerative nucleotide composition is sufficient to guarantee specific U2AF binding and spliceosome recruitment. We calculated the nucleotide usage near all variants of the 3′-splice sites ( Figs 3 , 5 , 7 and Supplementary Figs S11–S14 ). The comparison of these results with the corresponding thermodynamic profiles does not provide a direct answer because the nucleotide composition and its thermodynamic properties are interrelated. The thermodynamic stability of nucleotide duplexes has two components. The first component is the forces of the hydrogen interaction between complementary bases, and this component depends on the nucleotide composition. The second component is the stacking interaction between the bases, which depends mainly on the neighbouring di-nucleotide distribution. Therefore, the nucleotide distribution and its thermodynamic properties are interrelated. Although the sequence properties of the polypyrimidine region are known, the fact that they would lead to a specific DNA/DNA bias has been previously overlooked. The potential of the DNA/DNA bias to increase the accessibility of the PPT by preventing message/template annealing can enable the recruitment of U2AF65 to its preferred substrate [54] , and the two mechanisms may act in parallel to ensure assembly of the splicing machinery. Our study demonstrates that the least stable RNA/DNA duplexes as compared with the respective DNA/DNA duplexes are situated upstream from the 3′-splice site where the PPT is situated. This thermodynamic profile can prevent the re-annealing of mRNA to DNA to allow binding of U2AF65 to mRNA and initialize the primary steps of spliceosome assembly. This mechanism is supported by our results showing that annealing of antisense DNA oligonucleotides to a DNA/DNA-biased region inhibits pre-spiceosome complex A assembly. Genomes and annotations Annotations and sequences were obtained from the Ensembl genome browser [56] , [57] as follows: release 65 of H. sapiens genes (GRCh37.p5), release 68 of D. melanogaster genes (BDGP5), release 68 of D. rerio genes (Zv9) and release 68 of A. thaliana genes (TAIR 10). The full-length sequences of C. elegans transcripts were obtained from Wormbase (WB190). Sequences of 50 bp, flanking the transcript start sites, end sites and splice sites of C. elegans , were obtained from Ensembl (WB220). The list of trans -spliced C. elegans genes was taken from Allen et al . [58] Cryptic 3′-splice sites and their corresponding authentic 3′-splice sites were obtained from DBASS3 [33] . BP sequences were obtained from Gao et al . [37] Only BPs confirmed by a minimum of three lariat PCR with reverse transcription clones were considered. Pseudo exon and real exon data sets were obtained from Zhang et al . [40] Data sets for cassette exons, 3′-alternative splice sites, 5′-alternative splice sites and constitutive exons were obtained from HEXEvent database [32] . The retained intron data set was obtained from the UCSC Genome Table Browser [59] . Calculation of thermodynamic stability ΔG of the nearest-neighbour interactions was calculated by Perl-based software using Kowalski’s sliding-window approach [40] . Published values of ΔH and ΔS (at 37 °C and 1 M salt concentration) for each nearest-neighbour interaction for DNA/DNA duplexes [38] and RNA/DNA duplexes [39] were used. Calculations were carried out with a step size of 1 bp and a window size of 9 bp, except where specified otherwise. Colour-coded representation of the thermodynamic profiles was performed by Partek Genomics Suite software. The supporting web site ( http://bio21.bas.bg/ThermoHuman/ ) contains ΔG bias data for all human exon–intron junctions and the software used for DNA/DNA and RNA/DNA ΔG calculation. Mapping of potential BPs in H. sapiens We map the human BP consensus sequence yUn A y [37] at intronic sequence situated from 50th to 10th nucleotide upstream from 3′-splice site. High-resolution melting analysis Double-stranded cDNA of the wIL2, IL2 and eIL2 genes was amplified by PCR from plasmids pcDNA3-wIL2, pcDNA3-IL2 and pcDNA3-eIL2, respectively [12] . The RNA/DNA duplex of wIL2, IL2 and eIL2 was generated as follows: mRNA was produced by in vitro transcription by T7 RNA polymerase of the respective cDNA. Single-stranded DNA was produced by digestion with the lambda exonuclease (NEB) of a double-stranded PCR product with a 5′-phosphate attached to the strand that was to be removed. Finally, mRNA and template single-stranded DNA of the respective gene were annealed after initial denaturation and decreasing the temperature to 30 °C by steps of 1 °C. High-resolution melting analysis was performed using a Rotor-Gene 6000 instrument and Syto9 intercalating dye in 50 mM sodium phosphate buffer, pH 7.8, following the manufacturer’s instructions raising the temperature from 70 to 95 °C by 0.15 °C steps. Spliceosome complex formation in vitro assay Pre-spliceosome A complex assembly was carried out as described previously [55] , [60] . The 32P-UTP-radiolabelled RNA substrate (5′-gggaagcuugcugcacgucuagggcgcaguaguccaggg uuuccuugaugaugucauacuuauccugucccuuuuuuuuccacagCUCGCGGUUGAGGAC AAACUCUUCGCGGUCUUUCCAGUGGGGAUCC-3′), which includes 85 bp from the 3′-half of intron 1 and 46 bp of exon 2 of AdML transcript, was transcribed in vitro by T7 polymerase. Radiolabelled RNA substrate (20 fmol) and corresponding antisense DNA oligonucleotides (400 fmol) were annealed after initial denaturation and decrease of the temperature from 70 down to 36 °C by steps of 2 °C. ATP-depleted HeLa cell nuclear extract of 3 μl (IPRACELL) was combined with 13.3 mM HEPES (pH 8), 0.13 mM EDTA, 3 mM MgCl 2 , 24.9 mM KCl, 3.33% polyvinyl alcohol, 13.3% glycerol, 0.03% NP-40 and 0.66 mM dithiothreitol, supplemented with or without 2 mM ATP and 22 mM creatine phosphate, in a final volume of 9 μl. The mixture was incubated for 5 min at 30 °C. Heparin (1 μl; 10 mg ml −1 ) was added and incubated for 10 min at room temperature. The probe was loaded on a mini gel, composed of 0.5% agarose, 4% acrylamide, 0.05% bis-acrylamide, 50 mM Tris and 50 mM glycine. The gel was run for 2 h in 50 mM Tris and 50 mM glycine buffer. The gel was dried and exposed with a Kodak BioMax MR film or PhosphorImager screen. Statistics Spearman’s rank correlation nonparametric test with two-tailed significances was used to assess the relationship between ΔG and Tm of DNA/DNA or mRNA/DNA duplex stability of wil2, IL2 and eIL2 genes. Wilcoxon nonparametric rank-sum test was used to statistically evaluate the difference between two related samples: ΔG of DNA/DNA duplexes of intronic and exonic sequences of confirm C. elegans transcript ( n =10,961); ΔG of RNA/DNA duplexes of intronic and exonic sequences of confirm C. elegans transcript ( n =10,961). ΔG of RNA/DNA and DNA/DNA duplexes of intronic sequences of confirm C. elegans transcript ( n =10,961). Wilcoxon nonparametric rank-sum test was also used to statistically evaluate the thermodynamic profiles across splice sites. The analysis was performed as follows: we calculated the mean value of ΔG bias for the least stable region upstream from every 3′-spice site (situated between the 20th and the 2th nucleotide upstream from the 3′-splice site) and compared it with the mean value of the corresponding adjacent intronic sequence (situated between the 50th and the 21th nucleotide upstream from the 3′-splice site). We evaluated the differences between the two related samples ( H. sapiens , n =456,101; C. elegans , n =115,224). We calculated the mean value of ΔG bias for the most stable region of every 3′-spice site (situated between the 4th nucleotide of the intron and the 7th nucleotide of the exon from the 3′-splice site) and compared it with the mean value of the corresponding adjacent exonic sequence (situated between the 8th and the 50th nucleotide of the exons downstream from the 3′-splice site). We evaluated the difference between the two related samples ( H. sapiens , n =456,101; C. elegans , n =115,224). We calculated the mean value of ΔG bias for the most stable region of every 5′-spice sites (situated between the 8th nucleotide of the intron and the 8th nucleotide of the exon from the 5′-splice site) and compared it with the mean value of the corresponding adjacent exonic sequence (situated between the 9th and the 50th nucleotide of the exons downstream from the 5′-splice site). We evaluated the difference between the two related samples ( H. sapiens , n =456101; C. elegans , n =115,224). The differences between all pairs of related samples are statistically significant, with P -values <2e−15. How to cite this article: Nedelcheva-Veleva, M. N. et al . The thermodynamic patterns of eukaryotic genes suggest a mechanism for intron–exon recognition. Nat. Commun. 4:2101 doi: 10.1038/ncomms3101 (2013).